Slow cooling and efficient extraction of C-exciton hot carriers in MoS2monolayer In emerging optoelectronic applications, such as water photolysis, exciton fission and novel photovoltaics involving low-dimensional nanomaterials, hot-carrier relaxation and extraction mechanisms play an indispensable and intriguing role in their photo-electron conversion processes. Two-dimensional transition metal dichalcogenides have attracted much attention in above fields recently; however, insight into the relaxation mechanism of hot electron-hole pairs in the band nesting region denoted as C-excitons, remains elusive. Using MoS 2 monolayers as a model two-dimensional transition metal dichalcogenide system, here we report a slower hot-carrier cooling for C-excitons, in comparison with band-edge excitons. We deduce that this effect arises from the favourable band alignment and transient excited-state Coulomb environment, rather than solely on quantum confinement in two-dimension systems. We identify the screening-sensitive bandgap renormalization for MoS 2 monolayer/graphene heterostructures, and confirm the initial hot-carrier extraction for the C-exciton state with an unprecedented efficiency of 80%, accompanied by a twofold reduction in the exciton binding energy. Control of the relaxation behaviour of electron-hole pairs at the least possible cost is highly desirable for hot carrier-related optoelectronic applications [1] , [2] . In the field of bulk semiconductor photovoltaics, phonon-assisted hot-carrier cooling generates heat, so the maximum theoretical light-into-electricity conversion efficiency is limited to only ∼ 31% (ref. 3 ), a value that could double if all hot carriers could be extracted efficiently by suitable conductors [4] . To overcome this drawback, slowing down the hot-carrier relaxation via circumventing the phonon-assisted relaxation is the typical approach investigated [5] . Reducing the material dimensionality to achieve quantum confinement from one (two-dimensional material) to all three (quantum dot) dimensions is believed to slow hot-carrier cooling, since the enlarged energy spacing arising from quantum confinement causes a ‘phonon bottleneck’ [6] . Nevertheless, the initial hot-carrier extraction efficiency in typical quasi-zero-dimensional semiconductor quantum dot systems at room temperature is still low. For CdSe/CdS/ZnS core-shell quantum dots, only about a third of the photogenerated hot electrons located in the CdS shell will transfer to the electron acceptor (methyl viologen) [7] . Moreover, for bare CdSe quantum dots adsorbed within methyl viologen this hot electron extraction is negligible, because an extremely fast hot-carrier extraction process is required to compete against phonon-assisted relaxation [8] . Additional relaxation mechanisms that come into play are Auger-like processes and surface-state trapping, which are efficient in quantum dots [9] , [10] , unless the photogenerated electrons and holes are spatially separated to a certain extent [5] , [7] . Recently studied two-dimensional systems such as semiconducting transition metal dichalcogenides (TMDCs) with finite bandgaps [11] , [12] have been shown to be very promising for ultrathin and flexible energy conversion and storage devices [13] , [14] , [15] , [16] , [17] . Due to the parallel bands in their density of states or the so-called band nesting effect [18] , these atomically thin materials present strong optical responses even for excitation energies far exceeding their bandgaps. Recent work in atomically thin molybdenum disulfide (MoS 2 ) have suggested that the photoexcited electron-hole pairs in the ‘band nesting’ region (denoted as C-excitons) could exhibit a very fast intraband relaxation and a very slow indirect emission process due to spontaneous charge-separation in momentum space [19] , [20] . Hence, it can be expected that the resulting hot-carrier relaxation for the C-exciton state will be different from that associated with the band-edge excitons in atomically thin TMDCs. Moreover, because of the renormalized bandgap and enhanced electron-electron interactions induced by the reduced Coulomb screening [21] , as well as an indirect to direct bandgap transition attributed to the quantum confinement effect [22] , [23] in two dimensions, this C-exciton relaxation is expected to be distinguishable from its few-layer and bulk counterparts. Indeed, previous time-resolved studies have shown that the intervalley (K−Γ) transfer in MoS 2 bulk is very efficient due to the dominant indirect bandgap characteristic [24] , while for the few-layer MoS 2 case, although there is efficient charge carrier photogeneration [25] , the decay of neutral C-excitons is still faster than neutral band-edge excitons. However, the fundamental photophysical mechanism and detailed processes of hot-carrier relaxation and follow-up extraction for the C-exciton state in single-layer TDMCs have not yet been elucidated [26] , and could be crucial to understand the work mechanisms in related two-dimensional nanophotonic devices. In this article, we report the transient characteristics of the intrinsic high-energy C-exciton state in MoS 2 monolayer and MoS 2 monolayer/graphene heterostructure ( Fig. 1a ) by studying its femtosecond broadband transient absorption (TA) spectrum. We observe a slower hot-carrier relaxation for the C-excitons, in comparison with band-edge A/B-excitons, indicating the presence of an additional mechanism for the suppression of phonon-assisted relaxation which is not dominated by the quantum confinement effect. In combination with scanning tunnelling spectroscopic (STS) analysis and steady-state optical spectroscopies, we identify the screening-sensitive bandgap renormalization of single-layer MoS 2 with and without graphene as a substrate. The relevant initial charge transfer processes in MoS 2 monolayer/graphene heterostructures are confirmed, and a direct hot-carrier extraction with a remarkable efficiency of ∼ 80% is demonstrated for the C-exciton at room temperature, with corresponding values for A/B-excitons of 93%/81%. These results show that atomically thin TMDCs provide opportunities for modifying the electronic structure and manipulating the hot-carrier relaxation behaviour in two-dimensional d -electron systems. 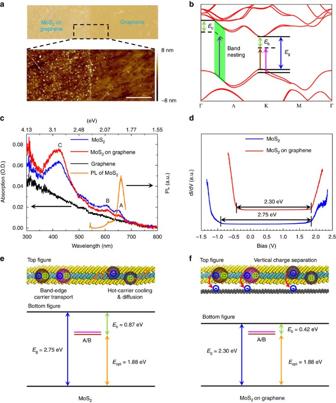Figure 1: Influence of graphene on the electronic bandgap of MoS2monolayer. (a) Optical microscope and AFM images of MoS2monolayer/graphene heterostructure. In the bottom, the scale bar is 2 μm. (b) Theoretically predicted energy band structure corresponding to the direct transitions in the momentum space of MoS2monolayers considering the spin-orbit coupling.Eg, energy gap;Eb, exciton binding energy. The green area is the band nesting region. The vertical brown, pink and purple arrows inbrepresent the optical transitions of A/B/C-exciton, respectively. (c) Steady-state absorption spectra of graphene, MoS2monolayer and MoS2monolayer/graphene heterostructure. O.D., optical density. The orange solid line is the PL spectrum of MoS2monolayer under 532 nm excitation. (d) STS spectra for MoS2monolayer and MoS2monolayer/graphene heterostructure. (e) Sketch of electronic and optical bandgaps for MoS2monolayer (bottom figure). The top image illustrates the MoS2monolayer (sky blue solid sphere represents the Mo atom, and yellow solid sphere represents the S atom); brown, pink and purple spheres represent the A/B/C-exciton, respectively; the orange curves represent the hot-carrier cooling and diffusion processes. (f) Sketch of electronic and optical bandgaps for MoS2monolayer/graphene heterostructure (bottom figure). The top illustration schematizes the MoS2monolayer/graphene heterostructure (black solid sphere represents the C atom); the red arrows indicate the vertical electron extraction processes.Eopt, optical bandgap. Figure 1: Influence of graphene on the electronic bandgap of MoS 2 monolayer. ( a ) Optical microscope and AFM images of MoS 2 monolayer/graphene heterostructure. In the bottom, the scale bar is 2 μm. ( b ) Theoretically predicted energy band structure corresponding to the direct transitions in the momentum space of MoS 2 monolayers considering the spin-orbit coupling. E g , energy gap; E b , exciton binding energy. The green area is the band nesting region. The vertical brown, pink and purple arrows in b represent the optical transitions of A/B/C-exciton, respectively. ( c ) Steady-state absorption spectra of graphene, MoS 2 monolayer and MoS 2 monolayer/graphene heterostructure. O.D., optical density. The orange solid line is the PL spectrum of MoS 2 monolayer under 532 nm excitation. ( d ) STS spectra for MoS 2 monolayer and MoS 2 monolayer/graphene heterostructure. ( e ) Sketch of electronic and optical bandgaps for MoS 2 monolayer (bottom figure). The top image illustrates the MoS 2 monolayer (sky blue solid sphere represents the Mo atom, and yellow solid sphere represents the S atom); brown, pink and purple spheres represent the A/B/C-exciton, respectively; the orange curves represent the hot-carrier cooling and diffusion processes. ( f ) Sketch of electronic and optical bandgaps for MoS 2 monolayer/graphene heterostructure (bottom figure). The top illustration schematizes the MoS 2 monolayer/graphene heterostructure (black solid sphere represents the C atom); the red arrows indicate the vertical electron extraction processes. E opt , optical bandgap. Full size image Steady-state optical characterization MoS 2 monolayers and graphene were grown by chemical vapour deposition (CVD) on SiO 2 /Si substrates and copper foils, respectively [27] , and then transferred to a fresh quartz substrate using a standard poly(methylmethacrylate) (PMMA) transfer method [28] . Details of MoS 2 monolayer and MoS 2 monolayer/graphene sample preparation and steady-state characterizations are presented in the Methods section. To confirm the sample quality, optical microscopy and atomic force microscopy studies, as well as steady-state photoluminescence (PL) and Raman characterization, were performed, as shown in Supplementary Figs 1−4 . Figure 1b,c exhibit, respectively, the ab initio calculation of the band structure related to the band nesting region for MoS 2 and the corresponding measured steady-state absorption and PL spectra. According to Fig. 1c , when MoS 2 monolayers are placed on a graphene substrate, the oscillator strengths of band-edge A/B-excitons around 650 and 600 nm decrease slightly, while for the high-energy C-exciton around 430 nm the oscillator strength increases. The resulting PL of the MoS 2 monolayer/graphene heterostructure (not shown) is found to be strongly quenched, in contrast to the reference case of MoS 2 monolayers alone ( Fig. 1c ), where the PL peak at around 660 nm (1.88 eV) is observed, corresponding to the optical bandgap ( E opt ) of the MoS 2 monolayer. These results imply complex interactions between the MoS 2 monolayer and substrates [29] that need to be understood. Electronic bandgap measurement and transient experiment To shed light on the correlations between the electronic structures of MoS 2 monolayer on different substrates and internal exciton relaxations, electronic bandgap and time-resolved ultrafast spectroscopy studies were performed. The influence of graphene on the electronic bandgap ( E g , equal to the quasiparticle bandgap, E q ) of MoS 2 monolayer is revealed by the STS analysis shown in Fig. 1d . It is found that E g is reduced from 2.75 eV for MoS 2 monolayer alone to 2.30 eV for MoS 2 monolayer/graphene heterostructure. Moreover, the measurements indicate that graphene lowers the conduction band minimum (CBM, left) of the MoS 2 monolayer by ∼ 0.45 eV, while the corresponding valence band maximum (VBM, right) is pinned at ∼ 1.85 eV below the Fermi level. The exciton binding energy, E b = E g – E opt , is calculated to be 0.42 and 0.87 eV for the MoS 2 monolayer with and without graphene, respectively. The former value approximates well to the previously reported values of E b of 0.48 eV and associated E g of 2.40 eV for CVD MoS 2 monolayers grown directly on cleaved graphite (HOPG) substrates [30] , and the latter is close to the reported theoretical predictions ( E b of 1.0 eV and E g of 2.8 eV) (refs 31 , 32 , 33 , 34 , 35 ). This indicates a screening-sensitive bandgap renormalization, similar to that reported for the MoSe 2 monolayer [21] . In addition, the reduced E b measured for MoS 2 monolayer/graphene heterostructures could facilitate the charge transfer from MoS 2 monolayer to graphene, as will be discussed later. The relevant energy levels for MoS 2 monolayer and MoS 2 monolayer/graphene heterostructure are presented in Fig. 1e,f , respectively, as extracted from the steady-state experimental data. According to our experimental observations and density functional theory (DFT) calculations ( Supplementary Fig. 5 ), the location of Dirac point of graphene in energy is close to the middle of bandgap of MoS 2 monolayer, about 1.20 eV higher than its VBM. The inherent excited-state relaxation processes for A/B/C-excitons in MoS 2 monolayers and MoS 2 monolayer/graphene heterostructures are elucidated by broadband TA experiments in transmission mode [36] , [37] . Typical TA spectra of MoS 2 monolayers under 400 nm excitation (pump density of 5 μJ cm −2 , initial exciton density of 1.28 × 10 12 cm −2 ) are shown in Fig. 2a . These spectra represent the pump-induced absorption changes observed in the samples, namely the differential optical density with and without pump light excitation (ΔO.D.=O.D. pump —O.D. w/o pump ). As it can be seen in Fig. 2a , there are three distinct negative transient species (bleaching signals) at around 656, 608 and 430 nm (1.89, 2.04 and 2.88 eV), corresponding to the energy states of A/B/C-excitons observed in the steady-state absorption spectrum ( Fig. 1c ), respectively. The positive peaks for atomically thin TMDCs as shown in Fig. 2a are usually attributed to peak shift and broadening of A/B/C-exciton states [38] , [39] , [40] ( Supplementary Fig. 6 and Supplementary Note 1 ), excited-state absorption and/or the absorption of new photogenerated transient species, for example, the effect of charges at high pump conditions [25] , [26] . 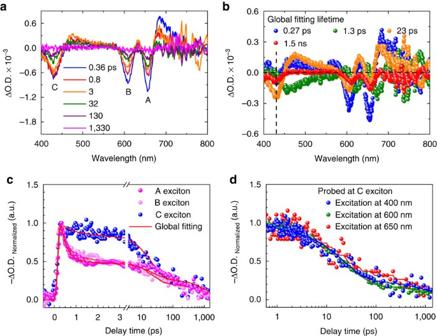Figure 2: Global fitting for transient absorption spectra of MoS2monolayers. (a) Transient absorption spectra of MoS2monolayers probed at different delay times under 400 nm excitation (pump density of 5 μJ cm−2, initial exciton density of 1.28 × 1012cm−2). (b) Global analysis for the transient absorption data ina. The vertical dashed line indicates the position of the C-exciton state, while the horizontal dashed line indicates ΔO.D.=0. (c) Normalized decay dynamics of A-, B- and C-exciton states under the pump condition ina. The red solid lines are the global fitting results. (d) Normalized decay dynamics of the C-exciton state under 400, 600 and 650 nm excitation with similar initial exciton density. The solid lines are the global fitting results. Figure 2: Global fitting for transient absorption spectra of MoS 2 monolayers. ( a ) Transient absorption spectra of MoS 2 monolayers probed at different delay times under 400 nm excitation (pump density of 5 μJ cm −2 , initial exciton density of 1.28 × 10 12 cm −2 ). ( b ) Global analysis for the transient absorption data in a . The vertical dashed line indicates the position of the C-exciton state, while the horizontal dashed line indicates ΔO.D.=0. ( c ) Normalized decay dynamics of A-, B- and C-exciton states under the pump condition in a . The red solid lines are the global fitting results. ( d ) Normalized decay dynamics of the C-exciton state under 400, 600 and 650 nm excitation with similar initial exciton density. The solid lines are the global fitting results. Full size image Through a global analysis [ΔO.D.= , where α i ( λ ) are the pre-exponential factors used for the calculation of decay-associated spectra (DAS), λ is probe wavelength and τ i are λ -independent lifetimes] (refs 37 , 41 ), as shown in Fig. 2b , it is deduced that there are at least four lifetime components for MoS 2 monolayers. For the band-edge bleaching region, the first two shortest lifetime components mainly represent the contributions of A/B-exciton populations. The lifetime component of 0.27 ps (blue) that is dominant in this spectral region could arise from fast nonradiative recombination, for example, exciton-exciton annihilation [42] , [43] , while the next lifetime component of 1.3 ps (green), since not only matches the spectral positions of steady-state PL peaks well, but also agrees with the fast decay component of band-edge emission [44] , it could be responsible for the radiative recombination of band-edge excitons. Concerning the bleaching region of the high-energy C-exciton state, the longer lifetime component of 23 ps (orange) is dominant, and could represent contributions of charge populations generated by self-separation of C-excitons in momentum space forming hot carriers. Finally, the remaining lifetime component in the nanosecond range (red) is used to match the long-lifetime decay background. It is therefore suggested that the global analysis on the TA data of MoS 2 monolayer should be applied when the initial exciton density is low enough, for example, less than 2 × 10 12 cm −2 adopted here. This analysis demonstrates a slower decay for the hot-carriers associated with the C-exciton state, especially at the first tens of picoseconds, as observed in Fig. 2c . It is worth noting that this anomalous relaxation behaviour is contrary to the expected faster decay for the C-exciton when considering only its electronic instability. In fact, the parallel bands in the density of states will induce very fast carrier relaxation, as we demonstrate in twisted bilayer graphene (see detailed discussions in Supplementary Figs 7,8 and Supplementary Note 2 ), where the average carrier lifetime is only ∼ 0.2 ps. However, for MoS 2 monolayers, in the case the excited-states of lower energy band-edge exciton states are already occupied, the C-exciton state under 400 nm excitation could cause a transient and complex excited-state Coulomb environment in the pump spectral region. In this context, the high-energy C-exciton relaxation in the band nesting region will slow down. To verify this hypothesis, we performed band-edge excitation TA experiments using 600/650 nm excitation ( Supplementary Fig. 9 ), for which the high-energy C-exciton state is still observed (that is, there is an efficient up-conversion process). For these band-edge excitation conditions, the initial exciton densities were set close to that for the 400 nm excitation case as presented in Fig. 2a-c . The global fitting results reveal subtle differences between the band-edge excitation and 400 nm excitation TA experiments (see detailed discussions in Supplementary Fig. 9 , Supplementary Note 3 ), suggesting a fast tunnelling mechanism from the high excited states of band-edge excitons to the C-exciton state [35] , which is consistent with our hypothesis ( Supplementary Fig. 10 and Supplementary Note 4 ). The resulting characteristic population decay dynamics for the C-exciton state generated by the different excitations give an average hot-carrier lifetime of 350±50 ps ( Fig. 2d ). TA experiments for higher exciton densities at 400 nm pump condition reveal another remarkable characteristic of the C-exciton state, which is an extremely weak initial exciton-density dependent relaxation. As shown in Fig. 3a , by increasing the pump density from 5 to 80 μJ cm −2 (initial exciton density ∼ 10 12 −10 13 cm −2 ), the initial TA signal amplitude of the C-exciton state probed at 0.36 ps increases and exhibits a linear behaviour even up to 240 μJ cm −2 ( Supplementary Fig. 11a ). Moreover, while the normalized decay traces at different pump densities for the C-exciton state show similar profiles ( Supplementary Fig. 11b ), the band-edge bound optical exciton states are strongly affected by the high initial exciton density (see detailed discussions in Supplementary Figs 12,13 and Supplementary Note 5 ). This implies a transient and reversible method to control the optical responses of band-edge excitons in ultrashort timescales [45] by changing the carrier population in the C-exciton state. 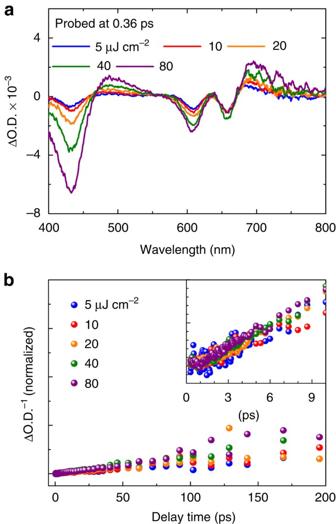Figure 3: Excitation-density dependent transient behaviours on MoS2monolayers. (a) Transient absorption spectra of MoS2monolayers probed at 0.36 ps under 400 nm excitation with different excitation power densities. (b) Reciprocal of decay traces of the C-exciton state (430 nm) under different excitation power densities, normalized at the minimum ΔO.D.−1. Inset shows the traces in the main panel within the first 10 ps. Figure 3: Excitation-density dependent transient behaviours on MoS 2 monolayers. ( a ) Transient absorption spectra of MoS 2 monolayers probed at 0.36 ps under 400 nm excitation with different excitation power densities. ( b ) Reciprocal of decay traces of the C-exciton state (430 nm) under different excitation power densities, normalized at the minimum ΔO.D. −1 . Inset shows the traces in the main panel within the first 10 ps. Full size image Free-carrier relaxation feature for C-exciton hot carriers Based on the rate equation [46] , describing the non-geminate/free carrier recombination, , where n 0 is the initial exciton density, t is time and k is the second-order rate constant for recombination, we find a linear relationship between ΔO.D. −1 at the C-exciton state and t in Fig. 3b . This linearity is consistent with a two-body recombination mechanism, and supports our hypothesis that photocarriers in the C-exciton state are hot carriers with free-carrier properties. In addition, this linearity is weakly dependent on the initial exciton density, which suggests that the exciton dissociation occurs efficiently in the C-exciton state, in agreement with the self-separation of photocarriers in the nesting region in momentum space. From linear fits using the rate equation at different pump densities, we estimate a second-order recombination rate constant of (3.8±0.2) × 10 −2 cm 2 s −1 at the extremely low initial exciton density limit ( n 0 →0) by extrapolating an exponential-decay phenomenological expression, as shown in Supplementary Fig. 11c . We now turn to the detailed description of hot-carrier relaxation processes in single-layer MoS 2 . It is well known in low-dimensional systems that many-body processes represent an important obstacle for achieving slow hot-carrier cooling. For the anomalous C-exciton relaxation in two-dimensional TMDCs, the band nesting effect is crucial, as it does not only provide an alternative high-energy exciton state, but also promotes self-separation of photocarriers in the nesting region in momentum space, which helps circumvent the Auger recombination channel owing to momentum mismatching. The quantum confinement in the two-dimensional system also changes the energy level alignment between the C-exciton and band-edge optical exciton (A/B-exciton) states. As the conduction and valence bands’ energy levels for the former are higher than those for the latter, hot carriers in the C-exciton state will eventually jump to the lowest energy states in momentum space. This process will then dominate over the indirect bandgap recombination that predominates in bulk and few-layers cases. Furthermore, when photoinduced band-edge excitons and their excited states generate C-excitons by an up-conversion/many-body process [26] , [35] , they also play a role in slowing down the C-exciton relaxation due to the transient excited-state Coulomb interactions [47] , [48] . By those factors together, a free-carrier recombination feature is created for the hot carriers in the C-exciton state of MoS 2 monolayer. Initial extraction process for C-exciton hot carriers Finally, we use the MoS 2 monolayer/graphene heterostructure to examine the initial carrier extraction processes. 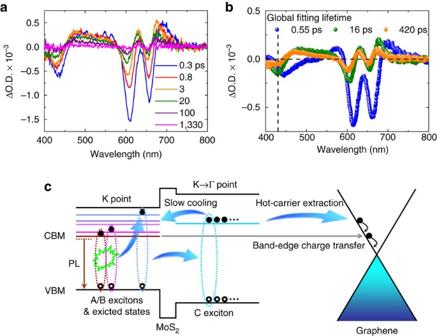Figure 4: Initial carrier extraction in MoS2monolayer/graphene heterostructure. (a) Transient absorption spectra of MoS2monolayer/graphene heterostructures probed at different delay times under 400 nm excitation (initial exciton density of 1.73 × 1012cm−2). (b) Global analysis for the transient absorption data ina. The vertical dashed line indicates the position of the C-exciton state, while the horizontal dashed line indicates ΔO.D.=0. (c) Illustration of the photophysical processes in the MoS2monolayer and initial charge transfer in the MoS2monolayer/graphene heterostructure. Figure 4a,b shows the TA spectra of MoS 2 monolayer/graphene films at room temperature (400 nm excitation, initial exciton density of 1.73 × 10 12 cm −2 ) and global fitting results, respectively. It is found that due to the influence of graphene, only three lifetime components compared to four previously are needed in the global analysis. Comparing with the results in bare MoS 2 monolayers, we calculate that the heterostructures present an initial carrier extraction efficiency of 93%, 81% and 80% for the A-, B- and C-exciton states, respectively. Detailed fitting data are presented in Supplementary Table 1 . The normalized dynamics of A-, B- and C-exciton states with and without the graphene substrate are also shown in Supplementary Fig. 14 . For the band-edge A-exciton, a high charge transfer efficiency (>90%) is expected, as reported in other atomically thin van der Waals heterojunctions [49] , [50] . In contrast, for the initial hot-carrier extraction in the C-exciton state, this is the first time to our knowledge that such a highly efficient hot-carrier transfer is demonstrated in the MoS 2 monolayer/graphene heterostructure. The related physical picture is illustrated in Fig. 4c . This observation could open new avenues for hot-carrier-driven optoelectronic applications [2] , such as water photolysis and singlet exciton fission based on atomically thin TMDCs, when other special electron acceptors are utilized to replace the graphene adopted here. Figure 4: Initial carrier extraction in MoS 2 monolayer/graphene heterostructure. ( a ) Transient absorption spectra of MoS 2 monolayer/graphene heterostructures probed at different delay times under 400 nm excitation (initial exciton density of 1.73 × 10 12 cm −2 ). ( b ) Global analysis for the transient absorption data in a . The vertical dashed line indicates the position of the C-exciton state, while the horizontal dashed line indicates ΔO.D.=0. ( c ) Illustration of the photophysical processes in the MoS 2 monolayer and initial charge transfer in the MoS 2 monolayer/graphene heterostructure. Full size image One novel transient feature found here is the slower carrier relaxation ( ∼ 350 ps) compared to the band-edge A/B-excitons, which stems from the favourable band alignment and complex excited-state Coulomb environment, rather than solely on quantum confinement in two-dimension systems. As a result, the hot-carrier relaxation in the C-exciton state is three orders of magnitude slower than the typical carrier relaxation for parallel bands in the density of states (such as ∼ 0.2 ps in twisted bilayer graphene). Thus, two lateral carrier transport modes in MoS 2 monolayers are revealed: slow hot-carrier diffusion and traditional band-edge carrier transport ( Fig. 1e , top), which are highly important for understanding the work mechanisms of two-dimensional optoelectronic devices based on TMDC monolayers [51] . It is worth noting that the hot-carrier diffusion in the C-exciton state of MoS 2 monolayer not only possesses the free-carrier relaxation feature, but also exhibits an initial-exciton-density-dependent second-order recombination rate constant. The latter could reflect the initial excited-state Coulomb environment around the photogenerated C-excitons. This contrasts with the band-edge free-carrier relaxation behaviour, such as in organometallic halide perovskite films [46] , where the second-order recombination rate constant is invariant under different pump fluences. In summary, our results establish a fundamental photophysical model in MoS 2 monolayers by carefully analysing the excited-state relaxation processes, especially the hot-carrier cooling and initial extraction for the C-exciton state in the band nesting region. A two-body recombination mechanism for the hot-carrier relaxation in the C-exciton state is proposed. In addition, an unprecedented initial hot-carrier extraction efficiency of 80% for the C-exciton state at room temperature is further identified when we use graphene as the electron acceptor (scheme in Fig. 1f , top). This highly efficient initial charge separation in the vertical direction occurred among the band-edge states (the initial carrier extraction efficiency is 93% and 81% for the band-edge A- and B-exciton states, respectively) and all high-energy excited-states indicates the optimized fabrication route for the construction of all two-dimensional van der Waals heterostructure devices. The heterostructure also yields a twofold reduction of E b in comparison with the pristine MoS 2 monolayer ( Fig. 1f , bottom). This further implies one approach to modulate the E g of single TMDC monolayer crystals by locally overlapping with other dielectric screening materials. Further theoretical research such as time-dependent quantum calculation is necessary for a better understanding of many-body processes involving the hot-carrier generation, relaxation and initial extraction in these atomically thin two-dimensional heterostructures. Sample preparation MoS 2 monolayers were grown by CVD on SiO 2 /Si substrates [27] . For the fabrication, the substrate was placed at the centre of the furnace, while the precursor powder (sulfur, 0.15 g) was placed in a quartz boat in a suitable upstream position. The smooth side of the SiO 2 /Si substrate was placed face down on a customized quartz half rod leaving a 2-μm gap between the substrate and the rod, and 0.05 g of MoO 3 was put on the back of the substrate. The quartz tube was heated from room temperature to 650 °C with inlet of 50-sccm Ar, and when the temperature reached the maximum value, the Ar flow was adjusted to 10 sccm. The furnace was kept for 20 min at 650 °C for the growth of MoS 2 . Uniform MoS 2 monolayers were obtained on the smooth side of the SiO 2 /Si substrate. For the MoS 2 transfer [28] , the MoS 2 film on Si wafer was first coated with a layer of PMMA (950 K, A3) by spin-coating (step 1: 500 r.p.m. for 10 s; step 2: 2,000 r.p.m. for 70 s), followed by annealing at 130 °C for 2 min. The PMMA at the edges of the SiO 2 /Si substrate was removed with a sharp blade to facilitate the following exfoliation of PMMA-capped MoS 2 from substrate. Then, a NaOH (3 mol l −1 ) solution at 100 °C was used to exfoliate the PMMA-capped MoS 2 from SiO 2 /Si. After that, the PMMA-supported MoS 2 film was transferred to deionized (DI) water so as to remove the etchant and residues. Fresh quartz substrates with and without graphene were then used to fish out the PMMA-capped MoS 2 film, followed by drying on a hot-plate (75 °C for 5 min and then 100 °C for 10 min). Hence, both MoS 2 monolayer and MoS 2 monolayer/graphene heterostructure samples were placed on quartz substrates. The PMMA was finally removed by acetone and the sample cleaned with isopropyl alcohol. Steady-state characterizations The optical imaging was performed in a Nikon Eclipse LV 100D system, and the atomic force microscopy imaging was performed by a BRUKER Dimension FastScan system using the tapping mode. The Raman/PL spectra and mapping were collected in a confocal system (The Alpha 300R). The wavelength of the excitation laser was 532 nm with a spot size of approximately 0.5 mm. The steady-state PL spectra and mapping were obtained with a 600 grooves mm −1 grating, while a 1,800 grooves mm −1 grating was used to get detailed line shapes of the Raman band. The steady-state absorption spectra were measured using a Shimadzu UV-2550 spectrophotometer. Scanning tunnelling microscopy (STM) measurements were carried out in an ultra-high vacuum system housing an Omicron LT-STM interfaced to a Nanonis controller. The sample was degassed overnight at 350 °C before STM/STS analysis was performed, and kept at 77 K during the measurements. For d I /d V spectra, the tunnelling current was obtained by a lock-in amplifier, with a modulation of 625 Hz and 40 mV. Note that the bias voltage ( V tip ) is applied on the STM tip; hence negative values correspond to the conduction band and positive values to the valence band. Femtosecond broadband transient absorption setup In the TA setup for both transmission and reflection modes, a mode-locked Ti:sapphire laser/amplifier system (Solstice, Spectra-Physics) was used (800 nm wavelength, 1.5-mJ pulse energy, 100 fs pulse width, 250 Hz repetition rate). The low frequency was set to allow matching of the signal with the collection system. The output of the amplifier was split into two parts, with the stronger beam used to generate the desired excitation light. For 600 and 650 nm excitation, a TOPAS system was adopted, while 400 nm excitation was directly doubled from 800 nm laser pulses. The broad-band white-light probe pulses from 400 to 850 nm generated from 2 mm thick water. The TA data were collected by a fibre-coupled spectrometer connected to a computer. The group velocity dispersion of the transient spectra was compensated by a chirp program. All the measurements were performed at room temperature. Theoretical calculations We performed the calculations using the DFT as implemented in the VASP codes. The exchange correlation energy was described by the generalized gradient approximation, in the scheme proposed by Perdew, Burke and Ernzerhof (PBE) (refs 52 , 53 ). A unit cell with vacuum region of 16 Å was used for the calculation, and a 9 × 9 × 1 Monkhorst-Pack mesh grid was used to sample the Brillouin zone. The cutoff energy of the plane wave basis was 520 eV. All atoms were relaxed until the Hellman-Feynman forces on individual atoms were less than 0.02 eV Å −1 . The effect of spin–orbit coupling was also included. Although the PBE calculation could underestimate MoS 2 ’s bandgap [54] , the resulting profile of energy band is expected to be correct. Data availability The data that support the findings of this study are available from the corresponding author on request. How to cite this article: Wang, L. et al . Slow cooling and efficient extraction of C-exciton hot carriers in MoS 2 monolayer. Nat. Commun. 8, 13906 doi: 10.1038/ncomms13906 (2017). Publisher's note: Springer Nature remains neutral with regard to jurisdictional claims in published maps and institutional affiliations.